Mapping causal links between prefrontal cortical regions and
            intra-individual behavioral variability Intra-individual behavioral variability is significantly heightened by
                aging or neuropsychological disorders, however it is unknown which brain regions are
                causally linked to such variabilities. We examine response time (RT) variability in
                21 macaque monkeys performing a rule-guided decision-making task. In monkeys with
                selective-bilateral lesions in the anterior cingulate cortex (ACC) or in the
                dorsolateral prefrontal cortex, cognitive flexibility is impaired, but the RT
                variability is significantly diminished. Bilateral lesions within the frontopolar
                cortex or within the mid-dorsolateral prefrontal cortex, has no significant effect
                on cognitive flexibility or RT variability. In monkeys with lesions in the posterior
                cingulate cortex, the RT variability significantly increases without any deficit in
                cognitive flexibility. The effect of lesions in the orbitofrontal cortex (OFC) is
                unique in that it leads to deficits in cognitive flexibility and a significant
                increase in RT variability. Our findings indicate remarkable dissociations in
                contribution of frontal cortical regions to behavioral variability. They suggest
                that the altered variability in OFC-lesioned monkeys is related to deficits in
                assessing and accumulating evidence to inform a rule-guided decision, whereas in
                ACC-lesioned monkeys it results from a non-adaptive decrease in decision threshold
                and consequently immature impulsive responses. In the context of cognitive tasks requiring rapid responding, the time
                taken to reach a decision and then select and execute an action, the response time
                (RT), reflects the efficiency of involved cognitive
                        functions [1] , [2] , [3] , [4] , [5] . The RT significantly
                fluctuates across trials even in highly trained individuals [3] , [4] , [5] , [6] . Such intra-individual trial-by-trial RT
                fluctuations might represent instabilities in the executive (cognitive) control of
                ongoing tasks. The RT variability might reflect weaker control, and/or lapse of
                attention and higher susceptibility to error commission. Indeed, a larger RT
                variability has been associated with occasional reduction in control or
                        attention [5] , [7] , [8] , [9] . Accumulated evidence indicates that the
                intra-individual RT variability is significantly exaggerated in
                        aging [1] , [6] , [8] , [10] , in neuropsychological disorders and patients
                afflicted with brain injuries [4] , [11] , [12] , [13] , [14] , [15] , and has even been shown to
                predict the all-cause mortality rate of the elderly [12] . Therefore, understanding
                the neural substrates and underlying mechanisms of intra-individual RT variability
                might bring critical insight into the pathophysiological processes that underpin
                lapses of attention and cognitive deficits that predispose afflicted people to
                accidents and social disadvantages. In line with the hypothesis that alterations in executive control and
                attention might underlie the trial-by-trial RT variability, imaging studies in
                humans have shown that activity in some of the main nodes of the attention and
                executive control networks such as the anterior cingulate cortex (ACC), posterior
                parietal cortex and dorsolateral prefrontal cortex (DLPFC), shows associations with
                RT and its trial-by-trial variability [5] , [7] , [16] . However, imaging studies
                have reported different, and even opposite, types of blood oxygen level-dependent
                (BOLD) signal change (increase, decrease, or temporal shift) in association with
                heightened RT variability. The negative and positive correlations between BOLD
                signals and RT variability have been associated with inadequate (low) levels of
                activation, and the compensatory recruitment of brain regions involved in cognitive
                control, respectively [5] , [7] , [16] , [17] , [18] , [19] , [20] . These differences might reflect the dynamic
                nature of the executive control of goal-directed behavior in which the role of
                neural circuits evolves in the course of consecutive trials: they might be involved
                in a kind of ‘preparatory set’ before the start of the
                        trial [9] , recruited by various cognitive functions within
                the trial, and also support post-trial learning and compensatory
                        processes [5] , [16] , [21] . The recruited neural processes and the level of
                their involvement might also differ depending on the task context e.g., the
                currently relevant rule or the decision outcome (correct or
                        error) [22] , [23] , [24] , [25] , [26] , [27] . Such dynamic changes might not be distinguished
                by the temporal resolution of current functional imaging techniques. Although imaging studies in humans indicate a link between neural
                activity in prefrontal and medial frontal regions and trial-by-trial alterations in
                        RT [1] , [2] , [3] , [5] , [7] , [10] , [14] , [16] , [19] , [20] , [28] , [29] , [30] , [31] , they do not necessarily
                establish causality between particular brain regions and such variabilities in the
                context of cognitive tasks. Neuropsychological examinations of patients with various
                neurodevelopmental and neuropsychological disorders or brain damage have brought
                important insights regarding the link between the integrity of certain brain regions
                and intra-individual RT variability [2] , [3] , [4] , [8] , [13] , however due to heterogeneity and inconsistency
                of lesion extent in patients and unilateral lesions in many cases, it has been
                difficult to delineate the causal role of particular prefrontal or medial frontal
                regions in intra-individual RT variability. Therefore, it is necessary to examine
                how selective and bilateral lesions (regional malfunction) in a particular brain
                region affect intra-individual RT variability in more highly controlled conditions. Macaque monkeys are suitable models for such an experiment, given the close
                similarity in the structure and organization of prefrontal and medial frontal
                regions between macaques and humans [32] , [33] , [34] , [35] and the fact that macaque
                monkeys can learn challenging cognitive tasks and perform hundreds of trials, which
                would enable reliable assessment of the intra-individual RT variability in a testing
                        session [36] , [37] , [38] . Moreover, unlike in
                patients with different lesions, groups of macaques with different lesions may have
                broadly similar pre-operative experience with behavioral tasks facilitating
                cross-group comparisons. Dominant models of decision-making [39] , [40] , [41] , [42] propose that the RT reflects three main
                processes: (1) evidence accumulation for a particular choice, which is reflected in
                the drift rate toward the decision threshold; (2) the decision threshold, which
                determines when evidence accumulation process ends and a response (rule-guided
                action) is delivered and (3) perceptual- and motor-related
                        processes [39] , [41] , [43] , [44] . In the context of the Wisconsin Card Sorting
                Test (WCST), the available evidence for the relevant rule changes trial by trial
                because of the imposed uncued rule changes as well as the decision feedback (reward
                and error-signal/no-reward given after correct and error trials, respectively). When
                evidence for the relevant rule is high, the accumulation of evidence (drift to the
                threshold) will occur faster and therefore the RT will be shorter. However, when
                evidence for the relevant rule is low, accumulation of evidence will necessarily
                take longer and lead to a longer RT. In this context, executive control would
                normally enhance the efficiency of evidence accumulation (increase the slope of
                drift), but its impairment/instability would disrupt evidence accumulation and
                appear as a longer RT and more errors. In parallel, alterations in decision
                threshold might also affect the RT so that an abnormally lower threshold will
                terminate evidence accumulation and lead to shorter RT but also to higher error
                likelihood. Psychophysical, functional imaging and modeling studies in humans
                suggest that both ACC and DLPFC are main nodes of an executive control network that
                supports evidence accumulation in the decision-making
                        process [39] , [41] , [43] , [44] . The involvement of this executive control
                network, and particularly ACC, in controlling impulsive responses (actions) have
                also been reported [39] , [41] , [43] . Related models propose that impulsive responses
                result from abnormal decrease in decision threshold, which might lead to a premature
                response before sufficient evidence accumulation [39] , [41] , [43] . This threshold change would manifest as a
                shorter RT but higher error likelihood [39] , [41] , [43] . To establish the causal relationship between specific brain regions and
                intra-individual RT variability, we made selective bilateral lesions in six distinct
                prefrontal and medial cortical regions in macaque monkeys performing a WCST analog,
                which is a challenging rule-guided decision-making task demanding cognitive
                flexibility to deal with frequently shifting rules [25] , [38] , [45] , [46] . In our WCST analog (henceforth referred to as
                WCST) (Fig. 1a ), the sample, the test items
                and their position were randomly changed trial-by-trial and there was no cue to the
                relevant rule or its frequent changes. Therefore, the monkeys had to find the
                relevant rule by trial and error and attain the rule-shift criterion (85% correct in
                20 consecutive trials) with each rule. Considering this task design and the fact
                that control monkeys could shift between rules (attain high performance following
                each rule shift) by committing a limited number of errors [25] , it is very unlikely that
                monkeys implemented an association-based strategy to adapt to frequent rule
                        shifts [33] . In addition, in earlier studies we showed that
                monkeys could generalize the rule to novel items [38] , which indicated they were
                applying a rule-based, but not association-based, strategy for action selection in
                the WCST. Previous lesion-behavioral studies with non-human primate models, in the
                context of the WCST analogs or set-shifting tasks, have shown the dissociable
                involvement of lateral, medial and orbital prefrontal regions in supporting
                cognitive flexibility in adapting to changing environments [25] , [47] , [48] , [49] , [50] . Neuronal activity
                recording and neuroimaging studies have shown that neural activities in a
                distributed network, including DLPFC, ACC, orbitofrontal cortex (OFC) and striatum,
                convey detailed information regarding rules and other task-related events in the
                WCST and set-shifting tasks [45] , [46] , [50] , [51] , [52] . Fig. 1: Computerized versions of the WCST and intended lesion
                                extent. a In the Wisconsin Card
                                Sorting Test (WCST), each trial commenced with sample onset at the
                                center of the screen and after monkeys touched the sample and
                                released their hand, three test items were presented on the left,
                                right and bottom of the sample. A correct application of the
                                matching rule led to the arrival of a reward. If monkeys did not
                                match based on the currently relevant rule (touched one of the
                                non-matching items) or did not respond within the response window,
                                an error signal was presented and no reward was delivered. b The schematic diagrams show the extent
                                of intended lesions in different groups of monkeys. Red regions show
                                the extent of intended lesion (all lesions were bilateral). The
                                details of lesion extent in each group are explained in the online
                                Methods section. The lesion extents were largely as planned as
                                assessed by microscopic inspection of post-mortem histological
                                sections (see Supplementary Information for figures and discussions
                                of lesion extent in individual animals) in all groups (except for in
                                the posterior cingulate cortex group wherein coronal magnetic
                                resonance images were inspected). Numerals: distance in mm from the
                                interaural plane. Full size image In the current study, selective lesions were made within DLPFC, ACC, or
                superior part of the dorsal-lateral prefrontal cortex (Fig. 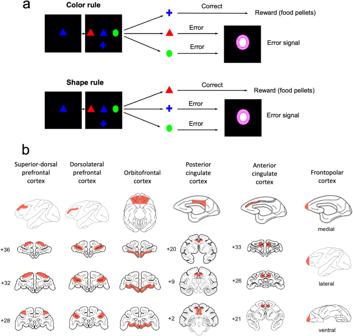Fig. 1: Computerized versions of the WCST and intended lesion
                                extent. aIn the Wisconsin Card
                                Sorting Test (WCST), each trial commenced with sample onset at the
                                center of the screen and after monkeys touched the sample and
                                released their hand, three test items were presented on the left,
                                right and bottom of the sample. A correct application of the
                                matching rule led to the arrival of a reward. If monkeys did not
                                match based on the currently relevant rule (touched one of the
                                non-matching items) or did not respond within the response window,
                                an error signal was presented and no reward was delivered.bThe schematic diagrams show the extent
                                of intended lesions in different groups of monkeys. Red regions show
                                the extent of intended lesion (all lesions were bilateral). The
                                details of lesion extent in each group are explained in the online
                                Methods section. The lesion extents were largely as planned as
                                assessed by microscopic inspection of post-mortem histological
                                sections (see Supplementary Information for figures and discussions
                                of lesion extent in individual animals) in all groups (except for in
                                the posterior cingulate cortex group wherein coronal magnetic
                                resonance images were inspected). Numerals: distance in mm from the
                                interaural plane. 1b ) (Table 1 ). These brain regions are critical nodes of the attention network
                in humans [24] , [26] , [53] , [54] . We also made selective bilateral lesions in the
                OFC (Fig. 1b ) because recent studies suggest
                that OFC might play crucial roles in the executive control of rule-guided behavior
                in the WCST and other set-shifting tasks [25] , [45] , [48] , [55] , [56] . In humans, posterior cingulate cortex (PCC) and
                frontopolar cortex comprise the main nodes of the default mode network. Resting
                state functional connectivity studies have suggested the presence of a comparable
                network in non-human primates, although the functional homology remains to be
                        established [57] , [58] , [59] , [60] . Imaging studies in humans
                have shown correlated activity change in these distributed brain networks in
                relation to the RT variability [5] , [10] , [16] , [18] , [19] , [28] , [30] , [61] , [62] . In this study, we also examined how selective
                lesions in OFC, frontopolar cortex and PCC affect the behavioral variability. Table 1 Demographic information about the two cohorts of monkeys in
                                this study Full size table Previous studies, in the context of WCST and other set-shifting tasks,
                have indicated that after rule or set shifts, macaque monkeys efficiently learn to
                adapt to the rule change by applying the currently relevant rule, however they
                continue to commit occasional errors indicating that despite long-term training with
                task switching, interference of the irrelevant rule affects their rule-based action
                        selection [25] , [38] , [63] , [64] . Therefore, we examined RT variability in
                correct (applying the relevant rule) or perseverative error (applying the irrelevant
                rule) trials, separately. In each daily testing session, the monkeys performed 300 trials and,
                with a shift criterion of 85% correct in 20 trials, they could attain the rule-shift
                criterion maximally 15 times in a daily session. Therefore, the total number of rule
                shifts in a daily session reflected the monkey’s cognitive flexibility in the day. To control the context in which decisions are made (i.e., the history of decision
                outcome: correct and error in preceding trials) we focused on correct trials
                that were preceded by correct trials (cC trials). We then calculated ‘coefficient of
                variability’ (Standard deviation/mean) for RT (RT-COV) in the second trial of each
                cC trial sequence (upper case letter). In perseverative error trials, the monkeys
                applied the irrelevant (previously relevant) rule. We selected perseverative error
                trials that were preceded by correct trials (cE trials) and calculated RT-COV in the
                second trial of each cE sequence. 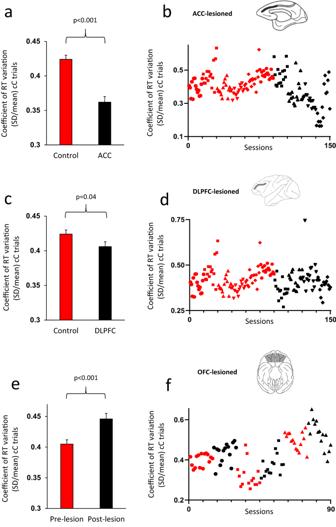Fig. 2: Selective lesions in the DLPFC, ACC or OFC modulate
                                    intra-individual response time (RT) variability. aThe coefficient of
                                    response time variability (RT-COV) was significantly smaller in
                                    the ACC-lesioned monkeys, compared to Control group
                                    (F(1140) = 35.66).bThe RT-COV
                                    of individual monkeys in 15 post-lesion sessions is shown for
                                    Control (red color) and ACC-lesioned monkeys (black color). The
                                    values for each monkey appear with a distinct marker shape.cThe RT-COV was
                                    significantly smaller in the DLPFC-lesioned monkeys, compared to
                                    Control group (F(1140) = 4.26).dThe RT-COV of individual monkeys in 15
                                    post-lesion sessions is shown for Control (red color) and
                                    DLPFC-lesioned monkeys (black color).eThe RT-COV is shown in the pre-lesion and
                                    post-lesion testing for the OFC-lesioned monkeys. RT-COV became
                                    significantly larger in the OFC-lesioned monkeys
                                    (F(1,42) = 12.56).fThe RT-COV
                                    of individual monkeys in 15 pre-lesion (red color) and 15
                                    post-lesion (black color) sessions is shown for OFC-lesioned
                                    monkeys. The cC sequence corresponds to a correct trial preceded
                                    by another correct trial. Data are presented as mean
                                    values ± SEM. Thepvalue
                                    shows the main effect of Lesion factor in the ANOVA. All
                                    comparisons were two-sided. Dorsolateral prefrontal cortex
                                    (DLPFC), anterior cingulate cortex (ACC), orbitofrontal cortex
                                    (OFC). Consequence of selective lesions in ACC When a nested ANOVA [Lesion-group (ACC/Control, between-subject
                    factor) × Monkey (10 monkeys, between-subject factor) nested within
                    Lesion-group] was applied to RT-COV in correct (cC) trials in ACC-lesioned and
                    Control monkeys, there was a highly significant effect of Lesion-group
                        (Table 2a ): the RT-COV was
                    significantly smaller in the ACC-lesioned group (Fig. 2a, b ), which was in contrast to the consequence of lesions
                    (larger RT-COV) in the PCC-lesioned monkeys (Fig. 3e ). Applying the ANOVA to SD values led to the same
                    conclusion (Table 2c and Fig
                        S 1a ). Despite a lower RT
                    variability, ACC-lesioned monkeys were significantly impaired in cognitive
                    flexibility: compared to control monkeys, ACC-lesioned monkeys achieved
                    significantly lower number of rule-shifts per daily session (Table 2h ), as has been reported in our previous
                            studies [25] . Table 2 Summary of behavioral changes following selective
                                    lesions Full size table Fig. 2: Selective lesions in the DLPFC, ACC or OFC modulate
                                    intra-individual response time (RT) variability. a The coefficient of
                                    response time variability (RT-COV) was significantly smaller in
                                    the ACC-lesioned monkeys, compared to Control group
                                    (F(1140) = 35.66). b The RT-COV
                                    of individual monkeys in 15 post-lesion sessions is shown for
                                    Control (red color) and ACC-lesioned monkeys (black color). The
                                    values for each monkey appear with a distinct marker shape. c The RT-COV was
                                    significantly smaller in the DLPFC-lesioned monkeys, compared to
                                    Control group (F(1140) = 4.26). d The RT-COV of individual monkeys in 15
                                    post-lesion sessions is shown for Control (red color) and
                                    DLPFC-lesioned monkeys (black color). e The RT-COV is shown in the pre-lesion and
                                    post-lesion testing for the OFC-lesioned monkeys. RT-COV became
                                    significantly larger in the OFC-lesioned monkeys
                                    (F(1,42) = 12.56). f The RT-COV
                                    of individual monkeys in 15 pre-lesion (red color) and 15
                                    post-lesion (black color) sessions is shown for OFC-lesioned
                                    monkeys. The cC sequence corresponds to a correct trial preceded
                                    by another correct trial. Data are presented as mean
                                    values ± SEM. The p value
                                    shows the main effect of Lesion factor in the ANOVA. All
                                    comparisons were two-sided. Dorsolateral prefrontal cortex
                                    (DLPFC), anterior cingulate cortex (ACC), orbitofrontal cortex
                                    (OFC). Full size image Fig. 3: Consequence of selective lesions in the sdlPFC, frontopolar
                                    cortex or PCC on intra-individual behavioral
                                    variability. a For sdlPFC-lesioned
                                    monkeys, there was no significant difference in RT-COV between
                                    the pre-lesion and post-lesion testing (F(1,42) = 0.96). b The RT-COV of individual
                                    monkeys in 15 pre-lesion (red color) and 15 post-lesion (black
                                    color) sessions is shown for sdlPFC-lesioned monkeys. The values
                                    for each monkey appear with a distinct marker shape. c For frontopolar-lesioned monkeys,
                                    there was no significant difference in RT-COV between the
                                    pre-lesion and post-lesion testing (F(1,56) = 0.082). d The RT-COV of individual monkeys in
                                    15 pre-lesion (red color) and 15 post-lesion (black color)
                                    sessions is shown for frontopolar-lesioned monkeys. e For PCC-lesioned monkeys, there was
                                    a significant difference in RT-COV between the pre-lesion and
                                    post-lesion testing, which appeared as a larger RT-COV
                                    (behavioral variability) following PCC lesion (F(1,42) = 30.31). f The RT-COV of individual
                                    monkeys in 15 pre-lesion (red color) and 15 post-lesion (black
                                    color) sessions is shown for PCC-lesioned monkeys. The p value and NS (Non-significant)
                                    indicate the main effect of Lesion factor in the ANOVA. Data are
                                    presented as mean values ± SEM. All comparisons were two-sided. Superior dorsal-lateral prefrontal cortex (sdlPFC), posterior
                                    cingulate cortex (PCC). Full size image When a two-way ANOVA [Response-type (cC/cE, within-subject
                    factor) × Monkey (6 monkeys)] was applied to RT-COV in cC and cE trials of the
                    Control group, the main effect of Response-type was highly significant (F(1,
                    84) = 61.05; P < 0.001, ηp2 = 0.42):
                    RT-COV was larger in cE (error) trials. Then, we examined the effects of the ACC
                    lesion on the RT variability difference between cC and cE trials. When a two-way
                    nested ANOVA [Lesion-group (ACC/Control) × Response-type (cC/cE, within-subject
                    factor) × Monkey (10 monkeys, nested within Lesion-group)] was applied to RT-COV
                    in cC and cE trials, there was a significant interaction between the
                    Response-type and Lesion-group factors (Table 2e ). The difference between cC and cE trials was smaller in
                    ACC-lesioned monkeys, which was mainly due to a reduced RT-COV in cE trials
                        (Fig. 4a ). The results were
                    consistent when we applied the ANOVA to SD values (Table 2f and Fig. S 4a ). Fig. 4: Consequence of selective brain lesions on behavioral
                                    variability in error trials. a − f The coefficient of response time variability
                                    (RT-COV) is shown in correct (cC) and error (cE) trials. a In ACC-lesioned monkeys,
                                    the RT-COV was decreased in both cC and cE trials, however the
                                    difference between cC and cE trials was significantly
                                    attenuated, which was mainly due to changes in cE trials
                                    (F(1140) = 4.25). b In
                                    DLPFC-lesioned monkeys, the RT-COV was decreased in both cC and
                                    cE trials, however the difference between cC and cE trials was
                                    not significantly affected (F(1140) = 1.42). c In OFC-lesioned monkeys, the RT-COV
                                    was significantly increased and the difference between cC and cE
                                    trials was significantly attenuated, however this was mainly due
                                    to changes in cC trials (F(1,42) = 7.80). d In sdlPFC-lesioned monkeys, there was no
                                    significant change in overall RT-COV or its difference between
                                    cC and cE trials (F(1,42) = 0.07). e In Frontopolar-lesioned monkeys, the RT-COV
                                    was significantly larger in error (cE) trials in both before and
                                    after the lesion, however the difference between cC and cE
                                    trials was not significantly affected (F(1,56) = 3.83). f In PCC-lesioned monkeys,
                                    the RT-COV was significantly larger in error trials in both
                                    before and after the lesion, however the difference between cC
                                    and cE trials was not affected (F(1,42) = 1.71). The p value shows the interaction
                                    between the Lesion and Response-type (cC/cE) factors in the
                                    ANOVA. Dorsolateral prefrontal cortex (DLPFC), anterior
                                    cingulate cortex (ACC), orbitofrontal cortex (OFC), superior
                                    dorsal-lateral prefrontal cortex (sdlPFC), posterior cingulate
                                    cortex (PCC). NS Non-significant. Data are presented as mean
                                    values ± SEM. All comparisons were two-sided. Full size image Consequence of selective lesions in DLPFC When the nested ANOVA was applied to RT-COV in cC trials in
                    DLPFC-lesioned and Control monkeys, the effect of Lesion-group was marginally
                    significant (Table 2a ): the RT-COV was
                    smaller in the DLPFC-lesioned group (Fig. 2c,
                        d ). Although the effect of Lesion-group was highly significant
                    with SD values: SD was smaller in the DLPFC-lesioned group (Table 2c and Fig. S 1b ), we have mainly considered the conclusion obtained with
                    RT-COV (marginally significant), because both the RT variability and mean RT
                    decreased in this case (see Methods, Data analyses). Despite a lower
                    RT-variability, DLPFC-lesioned monkeys showed significant impairment in adapting
                    to rule changes (Table 2h ) [25] . Regarding the difference in
                    fluctuations between cC and cE trials; there was no significant interaction
                    between the Response-type and Lesion-group factors with RT-COV
                        (Table 2e and Fig. 4b ), while the interaction was significant with
                    SD (Table 2f and Fig. S 4b ). Consequence of selective lesions in OFC To assess the effects of OFC lesion, we applied a two-way ANOVA
                    [Lesion (pre-lesion/post-lesion, within-subject factor) x Monkey (3 monkeys,
                    within subject factor)] to RT-COV of correct responses in the OFC group. There
                    was a highly significant main effect of Lesion factor (Table 2a ) without significant Lesion x Monkey
                    interaction (Table 2b ): the RT-COV in cC
                    trials became larger after OFC lesions (Fig. 2e,
                        f ). Applying the ANOVA to SD values also led to the same
                    conclusion (Tables 2 c and 2d and Fig. S 1c ). This result indicates that OFC-lesion led to a
                    remarkable increase in RT variability. There was a significant impairment in
                    cognitive flexibility after the OFC lesions (Table 2h ) [25] . As for the difference in RT
                    fluctuations between cC and cE trials, while the interaction between
                    Response-type and Lesion factors was significant with RT-COV (Table 2e and Fig. 4c ), there was no significant interaction with SD
                        (Table 2f and Fig. S 4c ). Consequence of selective lesions in sdlPFC When the two-way ANOVA was applied to RT-COV of correct responses
                    in the sdlPFC-lesioned group, there was no significant main effect of Lesion
                    factor (Table 2a and Fig. 3a ). Applying the ANOVA to SD values also led to
                    the same conclusion (Table 2c and Fig. S 1d ). The sdlPFC-lesioned monkeys
                    did not show any deficit in shifting between rules, either (Table 2h ) [25] . As for the difference in fluctuations
                    between cC and cE trials, there was no significant interaction between
                    Response-type and Lesion factors with RT-COV (Table 2e and Fig. 4d ),
                    while the interaction was marginally significant with SD (Table 2f and Fig. S 4d ). Consequence of selective lesions in the frontopolar cortex When the two-way ANOVA was applied to RT-COV of correct responses
                    in the frontopolar-lesioned group, there was no significant main effect of
                    Lesion-group (Table 2a and
                        Fig. 3c ). Applying the ANOVA to SD
                    values also led to the same conclusion (Table 2c and Fig. S 1e ). Lesions within the frontopolar cortex did not affect monkey’s ability in
                    shifting between rules either (Table 2h ) [65] . As for the difference in fluctuations
                    between cC and cE trials, there was no significant interaction between
                    Response-type and Lesion factors either with RT-COV (Table 2e and Fig. 4e ) or SD (Table 2f and Fig. S 4e ). Consequence of selective lesions in PCC When the two-way ANOVA was applied to RT-COV of correct responses
                    in PCC-lesioned group, there was a highly significant main effect of Lesion
                        (Table 2a ) without a significant
                    interaction (Table 2b ): the RT-COV
                    became significantly larger after PCC lesions (Fig. 3e ). With SD values, the main effect of Lesion was
                    significant but the interaction was also significant (Tables 2 c, and 2d ; and Fig. S 1f ). Although RT-COV was significantly increased in PCC-lesioned monkeys, they did
                    not show any significant deficit in cognitive flexibility in shifting between
                    rules (Table 2h ) [65] . As for the difference in fluctuations
                    between cC and cE trials, there was no significant interactions between
                    Response-type and Lesion factors either with RT = COV (Table 2e and Fig. 4f ) or SD (Table 2f and Fig. S 4f ). Figure 5 summarizes the
                    consequence of lesions on monkeys’ RT variability and cognitive flexibility
                    (number of rule-shifts) for all lesion groups. Fig. 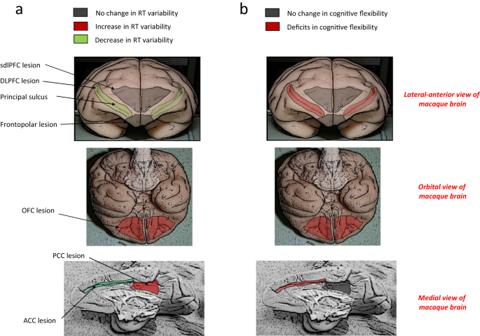Fig. 5: Dissociations in the involvement of six cortical regions in
                                    intra-individual RT variability. aThe effects of the
                                    bilateral lesion in different brain areas on the RT variability.
                                    Red and green colors indicate significant effects, which
                                    appeared as increased and decreased RT-COV, respectively. Gray
                                    color indicates no significant effect. All lesions were
                                    bilateral; however, the lesion extent is shown only on one
                                    hemisphere for ACC and PCC.bThe effects of the bilateral lesion in different areas on the
                                    cognitive flexibility. Red and gray colors indicate significant
                                    impairment and no deficits, respectively. Dorsolateral
                                    prefrontal cortex (DLPFC), anterior cingulate cortex (ACC),
                                    orbitofrontal cortex (OFC), superior dorsal-lateral prefrontal
                                    cortex (sdlPFC), posterior cingulate cortex (PCC). 5: Dissociations in the involvement of six cortical regions in
                                    intra-individual RT variability. a The effects of the
                                    bilateral lesion in different brain areas on the RT variability. Red and green colors indicate significant effects, which
                                    appeared as increased and decreased RT-COV, respectively. Gray
                                    color indicates no significant effect. All lesions were
                                    bilateral; however, the lesion extent is shown only on one
                                    hemisphere for ACC and PCC. b The effects of the bilateral lesion in different areas on the
                                    cognitive flexibility. Red and gray colors indicate significant
                                    impairment and no deficits, respectively. Dorsolateral
                                    prefrontal cortex (DLPFC), anterior cingulate cortex (ACC),
                                    orbitofrontal cortex (OFC), superior dorsal-lateral prefrontal
                                    cortex (sdlPFC), posterior cingulate cortex (PCC). Full size image Response time at different levels of evidence for rule-guided
                    actions To help infer the underlying mechanisms of RT variability, we
                    examined how the RT changed as the monkeys made multiple correct selections in
                    consecutive trials. 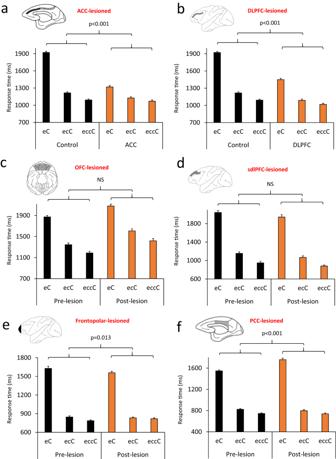Fig. 6: Response time (RT) at different levels of evidence for
                                    rule-guided actions. aMonkeys’ RT is shown
                                    in eC (a correct trial preceded by an error trial; e = error, C
                                    = correct), ecC and eccC trial sequences. RT was calculated in
                                    the current correct trial (upper case C) depending on the
                                    history (lower case letters). In Control monkeys, RT was the
                                    longest in eC trials, when the lowest level of evidence exists
                                    to guide rule-based action selection, however it was shorter in
                                    ecC and eccC trials. Compared to Control monkeys, ACC-lesioned
                                    monkeys had a shorter RT in all trial types (F(1140) = 105.69),
                                    however the difference in RT between Control and ACC-lesioned
                                    monkeys was the largest in eC trials (the lowest level of
                                    evidence).bA similar pattern
                                    of evidence-dependent modulation of RT was seen in the
                                    DLPFC-lesioned monkeys (F(1140) = 105.39).cEvidence-dependent modulation of RT was seen
                                    in OFC-lesioned monkeys, however their RT was longer at all
                                    evidence levels in the post-lesion testing (F(1,42) = 33.32).dEvidence-dependent
                                    modulation of RT was seen in sdlPFC-lesioned monkeys, however
                                    their RT was shorter at all evidence levels in the post-lesion
                                    testing (F(1,42) = 4.19). Evidence-dependent modulation of RT
                                    was seen in frontopolar-lesioned (F(1,56) = 0.86) (e) and PCC-lesioned monkeys
                                    (F(1,42) = 7.77) (f). Thepvalue shows the
                                    interaction between the Lesion and Evidence (eC/ecC/eccC)
                                    factors in the ANOVA. Data are presented as mean values ± SEM.
                                    All comparisons were two-sided. Dorsolateral prefrontal cortex
                                    (DLPFC), anterior cingulate cortex (ACC), orbitofrontal cortex
                                    (OFC), superior dorsal-lateral prefrontal cortex (sdlPFC),
                                    posterior cingulate cortex (PCC). We classified correct trials, according to the number of
                    correct trials preceding the current trial: The classification included eC
                    (correct trial immediately after an error trial), ecC (a correct trial preceded
                    by one correct trial after an error trial) and eccC (correct trial preceded by
                    two consecutive correct trials after an error trial) trials. We hypothesized
                    that monkeys’ RT will be the longest in eC trials, when the lowest level of
                    evidence exists to guide rule-based action selection, however monkeys’ RT would
                    be shorter in ecC and eccC trials because of accumulated evidence (receiving a
                    reward for a correct selection of rule) in these trials. We found that in the
                    Control monkeys the RT was the longest in eC trials, decreased in ecC trials,
                    and further decreased in eccC trials (the black bars of Fig. 6a , b ). We applied a multifactorial ANOVA [Evidence (eC/ecC/eccC, within-subject
                    factor) × Monkey (6 Control monkeys)] to the mean RT in each session. The main
                    effect of Evidence factor was highly significant (F(2168) = 945.15, P < 0.001, ηp2 = 0.92): the RT was
                    significantly longer in eC trials. Pairwise t tests (Bonferroni corrected) showed a significant difference between eC and ecC
                        ( p < 0.001), between eC and eccC
                        ( p < 0.001), and between ecC and
                    eccC trials ( p < 0.001). Fig. 6: Response time (RT) at different levels of evidence for
                                    rule-guided actions. a Monkeys’ RT is shown
                                    in eC (a correct trial preceded by an error trial; e = error, C
                                    = correct), ecC and eccC trial sequences. 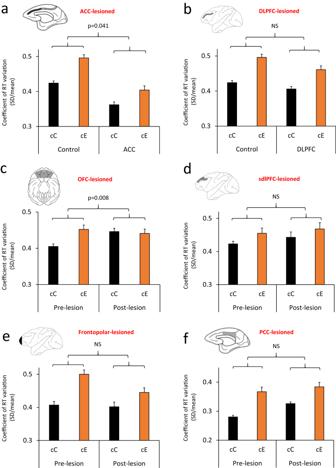RT was calculated in
                                    the current correct trial (upper case C) depending on the
                                    history (lower case letters). In Control monkeys, RT was the
                                    longest in eC trials, when the lowest level of evidence exists
                                    to guide rule-based action selection, however it was shorter in
                                    ecC and eccC trials. Fig. 4: Consequence of selective brain lesions on behavioral
                                    variability in error trials. a−fThe coefficient of response time variability
                                    (RT-COV) is shown in correct (cC) and error (cE) trials.aIn ACC-lesioned monkeys,
                                    the RT-COV was decreased in both cC and cE trials, however the
                                    difference between cC and cE trials was significantly
                                    attenuated, which was mainly due to changes in cE trials
                                    (F(1140) = 4.25).bIn
                                    DLPFC-lesioned monkeys, the RT-COV was decreased in both cC and
                                    cE trials, however the difference between cC and cE trials was
                                    not significantly affected (F(1140) = 1.42).cIn OFC-lesioned monkeys, the RT-COV
                                    was significantly increased and the difference between cC and cE
                                    trials was significantly attenuated, however this was mainly due
                                    to changes in cC trials (F(1,42) = 7.80).dIn sdlPFC-lesioned monkeys, there was no
                                    significant change in overall RT-COV or its difference between
                                    cC and cE trials (F(1,42) = 0.07).eIn Frontopolar-lesioned monkeys, the RT-COV
                                    was significantly larger in error (cE) trials in both before and
                                    after the lesion, however the difference between cC and cE
                                    trials was not significantly affected (F(1,56) = 3.83).fIn PCC-lesioned monkeys,
                                    the RT-COV was significantly larger in error trials in both
                                    before and after the lesion, however the difference between cC
                                    and cE trials was not affected (F(1,42) = 1.71). Thepvalue shows the interaction
                                    between the Lesion and Response-type (cC/cE) factors in the
                                    ANOVA. Dorsolateral prefrontal cortex (DLPFC), anterior
                                    cingulate cortex (ACC), orbitofrontal cortex (OFC), superior
                                    dorsal-lateral prefrontal cortex (sdlPFC), posterior cingulate
                                    cortex (PCC). NS Non-significant. Data are presented as mean
                                    values ± SEM. All comparisons were two-sided. Compared to Control monkeys, ACC-lesioned
                                    monkeys had a shorter RT in all trial types (F(1140) = 105.69),
                                    however the difference in RT between Control and ACC-lesioned
                                    monkeys was the largest in eC trials (the lowest level of
                                    evidence). b A similar pattern
                                    of evidence-dependent modulation of RT was seen in the
                                    DLPFC-lesioned monkeys (F(1140) = 105.39). c Evidence-dependent modulation of RT was seen
                                    in OFC-lesioned monkeys, however their RT was longer at all
                                    evidence levels in the post-lesion testing (F(1,42) = 33.32). d Evidence-dependent
                                    modulation of RT was seen in sdlPFC-lesioned monkeys, however
                                    their RT was shorter at all evidence levels in the post-lesion
                                    testing (F(1,42) = 4.19). Evidence-dependent modulation of RT
                                    was seen in frontopolar-lesioned (F(1,56) = 0.86) ( e ) and PCC-lesioned monkeys
                                    (F(1,42) = 7.77) ( f ). The p value shows the
                                    interaction between the Lesion and Evidence (eC/ecC/eccC)
                                    factors in the ANOVA. 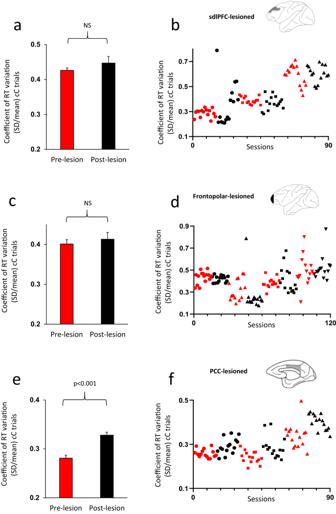Data are presented as mean values ± SEM. All comparisons were two-sided. Dorsolateral prefrontal cortex
                                    (DLPFC), anterior cingulate cortex (ACC), orbitofrontal cortex
                                    (OFC), superior dorsal-lateral prefrontal cortex (sdlPFC),
                                    posterior cingulate cortex (PCC). Fig. 3: Consequence of selective lesions in the sdlPFC, frontopolar
                                    cortex or PCC on intra-individual behavioral
                                    variability. aFor sdlPFC-lesioned
                                    monkeys, there was no significant difference in RT-COV between
                                    the pre-lesion and post-lesion testing (F(1,42) = 0.96).bThe RT-COV of individual
                                    monkeys in 15 pre-lesion (red color) and 15 post-lesion (black
                                    color) sessions is shown for sdlPFC-lesioned monkeys. The values
                                    for each monkey appear with a distinct marker shape.cFor frontopolar-lesioned monkeys,
                                    there was no significant difference in RT-COV between the
                                    pre-lesion and post-lesion testing (F(1,56) = 0.082).dThe RT-COV of individual monkeys in
                                    15 pre-lesion (red color) and 15 post-lesion (black color)
                                    sessions is shown for frontopolar-lesioned monkeys.eFor PCC-lesioned monkeys, there was
                                    a significant difference in RT-COV between the pre-lesion and
                                    post-lesion testing, which appeared as a larger RT-COV
                                    (behavioral variability) following PCC lesion (F(1,42) = 30.31).fThe RT-COV of individual
                                    monkeys in 15 pre-lesion (red color) and 15 post-lesion (black
                                    color) sessions is shown for PCC-lesioned monkeys. Thepvalue and NS (Non-significant)
                                    indicate the main effect of Lesion factor in the ANOVA. Data are
                                    presented as mean values ± SEM. All comparisons were two-sided.
                                    Superior dorsal-lateral prefrontal cortex (sdlPFC), posterior
                                    cingulate cortex (PCC). Full size image To assess the effects of ACC lesion, we applied a nested ANOVA
                        (Table 3 ) to the mean RT in each
                    session. The main effect of Lesion-group factor was highly significant
                        (Table 3a ): the RT was significantly
                    shorter in the ACC-lesioned group compared to the Control group. The main effect
                    of Evidence factor was also highly significant (Table 3b ): the RT was significantly longer in eC trials, but
                    decreased in ecC and eccC trials (Fig. 6a : ACC). The interaction between Lesion-group and Evidence
                    factors was also highly significant (Table 3c ): the RT difference between Control and ACC-lesioned
                    monkeys for eC was significantly larger than that for ecC or eccC trials
                        (Fig. 6a : ACC). Similar results were
                    also found for DLPFC-lesioned monkeys (Table 3 and Fig. 6b ). The
                    main effect of Evidence was significant in all lesion groups (Table 3b ). The main effect of Lesion factor was
                    significant in OFC-lesioned monkeys without a significant interaction between
                    Lesion and Evidence factors (Table 3b , c ), which indicates that RT was
                    longer in the post-lesion testing at all evidence levels. The Lesion effect was
                    also significant in sdlPFC monkeys without a significant interaction between
                    Lesion and Evidence factors (Table 3b , c ): RT was shorter at all evidence
                    levels. The main effect of Lesion was significant in PCC-lesioned, but not in
                    frontopolar-lesioned monkeys (Table 3a ). The interaction between Lesion and Evidence factors was significant in both
                    PCC-lesioned and frontopolar-lesioned monkeys (Table 3c ). Table 3 Results of analyses for changes in Response time (RT) at
                                    different levels of evidence Full size table RT variability was linked to the accuracy of upcoming decisions In our previous study [9] , we found that RT in humans and monkeys
                    was dependent on the accuracy of upcoming decision suggesting that
                    trial-by-trial changes in RT reflects fluctuations in the state of executive
                    control. To examine whether RT variability was linked to the accuracy in the
                    following trial (upcoming decision), we classified trials as cCc and cCe trials
                    (e = error; c = correct; cCc refers to three consecutive correct trials and cCe
                    refers to an error preceded by two consecutive correct trials). We calculated
                    RT-COV in the second trial of each sequence (which is denoted by upper case
                    letter). We applied a repeated-measure ANOVA [Trial-sequence (cCc/cCe,
                    within-subject factor) × Monkey (6 control monkeys)] to the RT-COV in each
                    session. The main effect of Trial-sequence was significant (F(1,84) = 5.77, p = 0.019, ηp2 = 0.06): the RT-COV was
                    higher in cCe trials. There was no significant interaction between
                    Trial-sequence and Monkey factors (F(5, 84) = 0.78, p = 0.56, ηp2 = 0.045). The higher RT variability in cCe trials
                    suggest that when the executive control state was at lower levels (i.e., the
                    likelihood of errors was higher in the following trial), the RT variability was
                    higher in correct trials. However, when we examined the effects of lesions in
                    ACC, DLPFC, sdlPFC, Frontopolar or PCC, there was no significant interaction
                    between Lesion and Trial-sequence factors in any lesion group (p > 0.35
                    for all lesion groups), which suggests that lesions in these brain regions did
                    not affect the difference in RT variability between cCc and cCe
                    sequences. We report dissociations in the involvement of different prefrontal and
                medial cortical regions in intra-individual RT variability. Dominant models, mainly
                emerging from studies in humans, propose that alterations in executive control and
                attention might underlie trial-by-trial RT variability: these models have suggested
                that heightened RT variability reflects weaker control, which might lead to lapses
                of attention and deficit in the task performance [3] , [5] , [10] , [14] , [16] , [18] , [19] , [28] , [30] , [31] , [62] . Here, mapping causal links between specific
                brain regions and intra-individual behavioral variability, we found that RT
                variability was significantly decreased in ACC-lesioned and in DLPFC-lesioned
                monkeys; and also accompanied by significant deficits in cognitive
                        flexibility [25] (Fig. 5 ). At first glance, these intriguing findings might appear
                contradictory to the predictions of models assuming direct associations between
                heightened RT variability and instability of executive control. However, our
                findings can be well explained in the broader context of decision-making processes
                in which RT reflects three main processes: (1) evidence accumulation for a
                particular choice, (2) the decision threshold, and (3) perceptual- and motor-related
                        processes [39] , [41] , [43] , [44] . In the context of cognitive tasks, RT might reflect various cognitive,
                sensory-motor and motivational aspects of behavior [3] , [5] , [16] . In a changing and complex environment, such as
                the WCST, where accumulation of evidence for available choices require executive
                control, the fluctuation of executive control will affect the rate of evidence
                accumulation and consequently correlate with RT fluctuations. In addition,
                alterations in decision threshold will also affect the RT and its fluctuation. In
                control (non-lesioned) animals, without changes in task contingencies, the
                sensory-motor processes would remain stable and therefore RT will mainly be
                associated with the rate of evidence accumulation and the decision threshold. In the
                context of the WCST, with its frequent uncued rule shifts, successful ongoing
                rule-guided behavior requires accumulation of evidence for the relevant rule by
                assessment of behavioral outcome (reward and
                        error/no-reward) [25] , [66] , by remembrance of the outcome of previous
                        trials [67] , by holding the memory of the currently relevant
                rule in working memory [38] , [46] , and by inhibiting the currently irrelevant
                        rule [32] , [33] , [68] , [69] . These processes are supported by executive
                control and therefore evidence accumulation processes would be dependent on the
                efficiency of executive control. In normal conditions, the efficiency and stability
                of executive control would be associated with the reduction in trial-by-trial RT
                        fluctuation [9] and with the ability of monkeys to shift between
                rules. In error trials, executive control might be weaker (unstable) and that would
                lead to a slower drift rate (Fig. S 3 ) and
                longer RT (Fig. S 5 ), disrupted links
                between RT and rule-guided behavior [9] , and eventually an erroneous action selection
                (lack of accumulated evidence for a rule). Our previous findings [25] indicate that basic perceptual- and
                motor-related processes remained intact in ACC-lesioned and DLPFC-lesioned monkeys
                because they did not show any impairment in control tasks where no shift in rules
                was required. Our findings (Fig. 6 ) suggest
                that the monkeys’ RT was significantly affected by the level of evidence accumulated
                following feedback to their choices. We have also previously reported that in
                Control (intact) monkeys, performance (percentage of correct responses) dropped to
                around 50% (chance level) following an error trial, however monkeys’ performance
                increased after the first correct (rewarded) trial and continued to improve
                following consecutive correct trials [25] . However, following lesions within ACC or
                DLPFC, monkeys’ performance increased more slowly following correct trials
                suggesting that ACC-lesioned and DLPFC-lesioned monkeys had impaired abilities in
                learning from consecutive rewards [25] , [52] . These results suggest that the executive
                control was significantly impaired and consequently led to difficulties in evidence
                accumulation in ACC-lesioned (and DLPFC-lesioned) compared to Control monkeys. 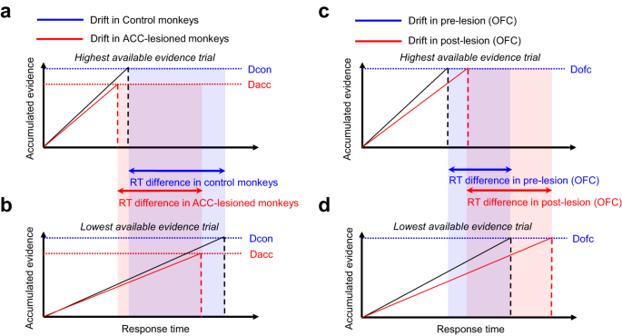Fig. 7: Drifting model predicting the consequence of lesions in ACC,
                                DLPFC and OFC on RT variability. The two cases of drifting model performance in which the
                                rate of evidence accumulation is the highest (a) and the lowest (b). The black and red oblique lines represent the
                                drift rate for Control and ACC-lesioned monkeys, respectively. The
                                explanation is given for ACC-lesioned monkeys, but can also be
                                considered for the DLPFC-lesioned monkeys. The abscissae and
                                ordinate represent the time and the amount of accumulated evidence
                                for a particular response, respectively. The model assumes that the
                                evidence for each response is accumulated constantly toward the
                                decision threshold and a response is made when the accumulated
                                evidence reaches the threshold. We assume that the decision
                                threshold is significantly lower in the ACC-lesioned monkeys (D-ACC:
                                red dotted line) as compared with that in the control monkeys
                                (D-control: blue dotted line). The distance between the two
                                same-color vertical lines indicates the magnitude of RT difference
                                (bidirectional horizontal arrows) within a session. The difference
                                depicted for the ACC-lesioned group (the light red region) is
                                smaller than the difference for the Control group (the light blue
                                region). This scheme is consistent with the results presented in
                                    Figs.2a and6a.cThe black and red oblique lines
                                represent the drift rate before and after OFC lesion, respectively
                                when the rate of evidence accumulation is the highest (c) and the lowest (d). Decision threshold in OFC-lesioned monkeys
                                (D-OFC) is shown with blue dotted line. We assume that the evidence
                                accumulation is significantly impaired after OFC lesion, which would
                                manifest as slower drift rates (red lines) at different levels of
                                available evidence, compared to the pre-lesion state (black lines).
                                The RT difference after OFC lesion (the light red region) is larger
                                than the difference before OFC lesion (the light blue region). This
                                scheme is consistent with the results presented in
                                    Figs.2e, and6c. Refer to
                                Supplemental material: ‘Computational background of Fig. 7’ for the
                                computational background. Dorsolateral prefrontal cortex (DLPFC),
                                anterior cingulate cortex (ACC), orbitofrontal cortex
                                (OFC). Figure 7a, b show the proposed scheme in
                which the accumulation of evidence is depicted as drifting lines (black and red
                lines in Control and ACC-lesioned monkeys, respectively) progressing toward the
                theoretical decision threshold (blue and red horizontal dotted lines in Control and
                ACC-lesioned monkeys, respectively). In the context of the WCST, when the available
                evidence for a rule is high (Fig. 7a ), the
                process of evidence accumulation would proceed rapidly leading to a fast response
                (marked by vertical dashed lines); but when the available evidence for a rule is low
                    (Fig. 7b ), the evidence accumulation
                would require a longer time and therefore lead to a longer RT. Fig. 7: Drifting model predicting the consequence of lesions in ACC,
                                DLPFC and OFC on RT variability. The two cases of drifting model performance in which the
                                rate of evidence accumulation is the highest ( a ) and the lowest ( b ). The black and red oblique lines represent the
                                drift rate for Control and ACC-lesioned monkeys, respectively. The
                                explanation is given for ACC-lesioned monkeys, but can also be
                                considered for the DLPFC-lesioned monkeys. The abscissae and
                                ordinate represent the time and the amount of accumulated evidence
                                for a particular response, respectively. The model assumes that the
                                evidence for each response is accumulated constantly toward the
                                decision threshold and a response is made when the accumulated
                                evidence reaches the threshold. We assume that the decision
                                threshold is significantly lower in the ACC-lesioned monkeys (D-ACC:
                                red dotted line) as compared with that in the control monkeys
                                (D-control: blue dotted line). The distance between the two
                                same-color vertical lines indicates the magnitude of RT difference
                                (bidirectional horizontal arrows) within a session. The difference
                                depicted for the ACC-lesioned group (the light red region) is
                                smaller than the difference for the Control group (the light blue
                                region). This scheme is consistent with the results presented in
                                    Figs. 2 a and 6a . c The black and red oblique lines
                                represent the drift rate before and after OFC lesion, respectively
                                when the rate of evidence accumulation is the highest ( c ) and the lowest ( d ). Decision threshold in OFC-lesioned monkeys
                                (D-OFC) is shown with blue dotted line. We assume that the evidence
                                accumulation is significantly impaired after OFC lesion, which would
                                manifest as slower drift rates (red lines) at different levels of
                                available evidence, compared to the pre-lesion state (black lines). The RT difference after OFC lesion (the light red region) is larger
                                than the difference before OFC lesion (the light blue region). This
                                scheme is consistent with the results presented in
                                    Figs. 2 e, and 6c . Refer to
                                Supplemental material: ‘Computational background of Fig. 7’ for the
                                computational background. Dorsolateral prefrontal cortex (DLPFC),
                                anterior cingulate cortex (ACC), orbitofrontal cortex
                                (OFC). Full size image Importantly, we propose that the decision threshold was significantly
                lower in ACC-lesioned monkeys and probably DLPFC-lesioned monkeys as well (compared
                to Control monkeys) and consequently led to earlier termination of evidence
                accumulation and culmination in impulsive responses, which would also increase the
                error likelihood. Therefore, alterations in RT will be accompanied by more errors in
                the rule selection. A lower decision threshold also explains a reduction in RT
                variability. Figure 7 shows the rate of
                evidence accumulation at the highest (Fig. 7a ) and the lowest (Fig. 7b ) for Control and ACC-lesioned monkeys. In line with our
                findings (Fig. 6a ); the RT was shorter in
                ACC-lesioned monkeys as compared with Control monkeys both at the highest and lowest
                levels of evidence. In addition, the RT variability (difference in RT between the
                highest and lowest levels of evidence) was smaller in ACC-lesioned monkeys as
                compared with Control monkeys. The distance between the two same-color vertical
                lines indicates the magnitude of RT difference within a session. The difference
                depicted as the red shadow for the ACC-lesioned group is smaller than the difference
                depicted as the blue shadow for the Control group (Fig. 7a, b ). Thus, our proposed scheme predicts that, in the
                ACC-lesioned monkeys, the within-session RT variability would be significantly
                smaller compared to the Control monkeys because of the lower decision threshold
                (also see the Supplementary material). In fact, we found significant decrease in RT
                variability in ACC-lesioned (Fig. 2a ) and
                marginally significant decrease in DLPFC-lesioned monkeys (Fig. 2c ), which was accompanied by significant deficit in
                cognitive flexibility in the WCST [25] . In our conclusions regarding the decrease in RT variability and its
                underlying mechanisms, we have mainly focused on ACC-lesioned monkeys because the
                effects of ACC lesion were highly significant. We have previously reported that
                Control (intact) monkeys showed RT slowing in error trials (compared to the correct
                trials) and this error-slowing appeared regardless of the preceding trial (correct
                or error) [52] . The error slowing might reflect weaker control and the associated higher level of
                uncertainty in error trials [9] . However, error slowing was significantly
                attenuated in ACC-lesioned monkeys [52] , which might be related to the lower
                decision threshold that led to a faster response despite lack of enough accumulated
                evidence. We found that RT variability was significantly larger in error (cE)
                compared to correct (cC) trials (Fig. 4a ). Figures S3a and S3b show evidence accumulation (two drift lines at
                two evidence levels) for Control and ACC-lesioned monkeys in correct and error
                trials, respectively. Our scheme predicts that the RT difference (the horizontal
                bidirectional arrow connecting the two vertical dashed lines) in correct trials
                (Fig. S 3a ) will be smaller than that in
                error trials (Fig. S 3b ) for both Control
                and ACC-lesioned monkeys (see the Supplementary material). The proposed scheme also
                predicts that the decrease in decision threshold, which might occur in ACC-lesioned
                monkeys, would lead to a smaller RT variability in ACC-lesioned monkeys in both
                correct (Fig. S 3a ) and error trials (Fig. S 3b ), which are supported by our
                observations (Fig. 4a ). Our scheme also
                predicts that the lower decision threshold in the ACC-lesioned monkeys would lead to
                a smaller difference in RT variability between correct and error trials, as compared
                with the difference in the control monkeys. If the rate of evidence accumulation is
                constant over the time, namely, the drifting line is straight, the ratio of the
                magnitude of the RT variability is proportional to the ratio of the decision
                threshold for both correct (Fig. S 3a ) and
                error (Fig. S 3b ) trials (see the
                Supplementary material). In fact, our findings support this scheme by showing that
                the difference in RT variability between correct and error trials was significantly
                attenuated in ACC-lesioned monkeys (appeared as a significant interaction between
                Response-type and Lesion factors) (Fig. 4a ). The pattern of behavioral changes in the OFC-lesioned monkeys was
                unique among all lesion groups in that they showed a significantly higher level of
                RT variability (Fig. 2e ), which was
                accompanied by remarkable deficits in cognitive flexibility (Table 2h ) [25] . These indicate that the behavioral effects
                of OFC lesions were in stark contrast to the consequence of lesions in ACC
                suggesting that OFC plays a distinctly different role in RT variability, and
                presumably in trial-by-trial adjustment of executive control. In the frame of
                drifting model schema, we assume that the rate of evidence accumulation became lower
                after OFC lesion, at both the highest and lowest levels of evidence
                    (Fig. 7c, d ). In line with our findings
                    (Fig. 6c ); at both the highest and
                lowest levels of evidence, the RT was longer after OFC lesion (Fig. 7c, d ). The reduced rate of evidence accumulation at
                various levels of evidence will also lead to higher RT variability (larger
                difference in RT between various levels of evidence) in OFC-lesioned monkeys
                    (Fig. 7c, d , and the Supplementary
                material), which was what we observed (Fig. 2e ). Different lines of evidence suggest that OFC is crucially
                involved in the executive control of rule-guided behavior in humans and
                        monkeys [25] , [45] , [49] , [56] , [70] , [71] , [72] , [73] . Neuronal activity in OFC
                is also associated with monkeys’ RT and accuracy in the upcoming decisions, which
                suggests that OFC might be involved in setting the executive control and restoring
                its allocation based on the behavioral outcome [9] , [72] . Importantly, OFC lesions disrupt behavioral
                improvement following reward, which suggests that OFC is crucially involved in
                evidence accumulation for the relevant rule by assessing the decision
                        outcome [25] , [48] . In our proposed scheme, these contributions of
                OFC to executive control will enhance evidence accumulation for the relevant rule. Therefore, the significant increase in RT variability (Fig. 2e ), and the deficit in cognitive
                        flexibility [25] , in OFC-lesioned monkeys, might be related to
                the impaired executive control and consequently lack of support for assessing and
                accumulating evidence for proper rule-guided decisions. Having observed the effects of damage to the executive control network
                (such as ACC and DLPFC), we examined how selective lesions within frontopolar cortex
                or PCC affect RT variability. These two regions are main nodes of the default mode
                network in humans [61] and might also have corresponding roles in
                non-human primates [57] , [58] , [59] , [60] . Intriguingly, the effects
                of lesions differed between frontopolar cortex and PCC lesions in that RT
                variability was significantly increased in PCC-lesioned monkeys (Fig. 3e ), but not in the frontopolar-lesioned monkeys
                    (Fig. 3c ). Lesions in frontopolar cortex
                or PCC did not affect monkeys’ ability in shifting between rules (Table 2h ) [65] . Although the role of default mode network
                and its neural substrate in non-human primates remain to be
                        established [57] , [58] , [59] , [60] , [61] , these findings bring
                insights regarding dissociations in contribution of the neural nodes, within the
                default node network and also between the executive control and default mode
                networks, to RT variability. There were also remarkable dissociations in
                contribution of anterior (ACC) and posterior (PCC) cortical regions of the cingulate
                sulcus to the trial-by-trial RT variability: lesions in ACC decreased RT variability
                    (Fig. 2a ) and the difference in RT
                variability between cC and cE trials (Fig. 4a ), but PCC lesions increased RT variability (Fig. 3e ) with no effect upon the difference between
                correct and error trials. Intra-individual RT variability is predictive of individual’s survival
                and has been considered as a behavioral biomarker of brain injury and wide-ranging
                neuropsychological disorders; moreover, RT variability might even appear earlier
                than most other diagnosable symptoms. However, it has been difficult to link such
                changes to malfunctions of particular brain regions. Here, in an extensive
                lesion-behavioral study in macaque monkeys in the context of a challenging
                rule-shifting task, we mapped the causal link between various different brain
                regions and intra-individual RT variability and found remarkable functional
                dissociations between the neural nodes of distributed executive control network
                (ACC, DLPFC, OFC), PCC and frontopolar cortex (Fig. 5 and Table 2 ). Our
                findings indicate that both extremes of RT variability (significant decrease or
                significant increase) might be associated with cognitive deficits in goal-directed
                behavior. The exaggerated RT variability in patients afflicted with traumatic brain
                injury or neuropsychological disorders might not be related to the selective
                malfunction of ACC because selective lesion in ACC was found to decrease RT
                variability. In addition, lesions in frontopolar cortex or sdlPFC do not affect RT
                variability. Selective lesions in OFC or in PCC led to significant increases in RT
                variability; however, only OFC-lesioned monkeys showed concomitant increase in RT
                variability and deficits in cognitive flexibility (Fig. 5 ). RT variability is exaggerated in aging [8] , [10] and age-related changes in cognitive
                flexibility has been reported in humans and monkeys [74] , [75] . Early damage to prefrontal cortex or its
                broader network might also affect cognitive flexibility [76] , [77] . Our study examined RT variability and the
                effects of selective lesions in adult monkeys and found significant dissociations in
                contribution of frontal regions to RT variability. Future studies examining RT
                variability in aged non-human primate models might help to delineate the underlying
                mechanisms of age-related RT changes and concomitant cognitive declines. Furthermore, investigating the early-onset damage to prefrontal cortical regions
                might bring further insights regarding the developmental changes in RT variability
                and the contribution of prefrontal cortical regions [77] , [78] . Our findings in non-human primate models
                have great translatability to understand the neural basis of behavioral variability
                in humans, however direct generalization of our findings to human population needs
                to be done cautiously considering that our study was conducted in a limited number
                of monkeys to minimize the animal use, and that a long-term training (about 1 year
                for each monkey) was required to learn performing the WCST. We conclude that OFC has a unique contribution to RT variability and
                associated cognitive deficits, which might be related to its crucial role in
                assessing the behavioral outcome and adjusting evidence accumulation for making
                effective rule-guided decisions. This interpretation is also supported by previous
                studies in non-human primates indicating the crucial role of OFC in assessing the
                behavioral outcome and in shifting between rules and
                        strategies [45] , [48] , [56] , [70] , [71] , [72] , [73] , [79] . Previous studies [25] , [32] , [80] , [81] , [82] have ascribed various
                critical functions for ACC in executive control of goal-directed behavior, such as
                monitoring demands (conflict, uncertainty) for allocation of control and assessing
                the outcome of actions. Our findings support the possibility of impairments in these
                functions, which would adversely affect evidence accumulation in the context of
                WCST; however, we propose that concomitant decrease in decision threshold in
                ACC-lesioned monkeys is the most parsimonious explanation of our findings, because
                it consistently explains the decrease in RT variability and other aspects of their
                behavior in the WCST. This scheme also conforms well with previous findings in
                humans showing that impulsive responses with higher error likelihood, as manifested
                in some neuropsychological disorders, might be linked to ACC
                        dysfunction [41] , [83] . Previous studies [47] , [48] , [74] , [84] , examining the consequence of lesions in
                monkeys’ prefrontal cortex, have mainly focused on alterations in mean RT and
                accuracy (% correct/error), however our findings suggest that RT variability might
                be significantly and distinctively affected by malfunction of specific frontal
                cortical regions. Re-examining the RT variability in these studies might bring
                further insight to the underlying mechanisms of associated behavioral deficits. Our
                findings in monkeys take a significant step toward understanding the causal link
                between the function of particular brain regions and intra-individual RT variability
                in the context of goal-directed behavior and may bring critical insights to the
                neural substrate and pathophysiological mechanisms that underlie altered response
                variability and related cognitive deficits in patients afflicted with brain damage
                or neuropsychological disorders. Study design and lesion groups Macaque model 21 macaque monkeys (7 macaca
                            fuscata and 14 macaca
                            mulatta ) were trained to perform a computerized analog
                        version of the WCST. Seven monkeys in the first cohort of animals were
                        trained, operated and tested at Oxford University and the rest of studies
                        were conducted at RIKEN institute. Table 1 includes demographic information (sex, species) of all
                        21 monkeys. The effects of lesions on the ability of
                                ACC-lesioned [25] , [52] , DLPFC-lesioned [25] ,
                                OFC-lesioned [25] , [45] ,
                                frontopolar-lesioned [65] and
                                PCC-lesioned [65] monkeys in shifting between rules
                        (cognitive flexibility) have been reported in our previous
                                publications [25] , [42] , [50] , [63] . All experimental procedures in Japan
                        conformed to the ethics guidelines specified by RIKEN Center for Brain
                        Science. All experimental procedures at Oxford University followed the
                        guidelines of the UK Animals (Scientific Procedures) Act of 1986, licensed
                        through the UK Home Office, and approved by Oxford University Committee on
                        Animal Care and Ethical Review. In the first cohort of macaque monkeys, 14 monkeys were trained
                        to perform a computerized version of the WCST (Fig. 1a ). Then, based on individuals’ pre-lesion
                        performance (mean number of rule-shifts in each testing session), the
                        monkeys were assigned to three separate groups of matched abilities. The
                        range and mean of the numbers of pre-lesion shifts between rules were
                        comparable between groups. In one group of 4 monkeys, bilateral lesions were
                        made in both banks and fundus of principal sulcus on the lateral surface of
                        prefrontal cortex (DLPFC group) (Figs. 1b and S 6 ), in
                        another group of 4 monkeys, bilateral lesions were made within ACC (ACC
                        group) (Figs. 1b and S 6 ), but the other 6 monkeys (Control group)
                        did not receive any lesion and remained as unoperated controls. Monkeys’
                        performance in the 15 post-lesion sessions was compared between the lesioned
                        and control groups. A two-week rest was considered after the lesion
                        operation for all groups. Unoperated control (intact) monkeys also rested
                        for 2 weeks between pre-lesion and post-lesion testing. In the second stage
                        of the study, the 6 aforementioned Control monkeys were assigned to two
                        performance-matched lesion groups. In three monkeys, bilateral lesions were
                        made within the OFC (OFC group) (Figs. 1b and S 7 ) and
                        in the other three monkeys, bilateral lesions were made within superior part
                        of the dorsal-lateral prefrontal cortex (sdlPFC group) (Figs 1b and S 7 ). For the OFC and sdlPFC groups, the consequence of
                        lesions was examined by comparing monkeys’ behavior between 15 pre-lesion
                        testing sessions and 15 post-lesion sessions. Monkeys in the OFC and sdlPFC
                        groups had performed more sessions compared to the ACC and DLPFC groups. However, the effects of lesions within the OFC or in the sdlPFC on
                        behavioral measures were assessed by comparing the pre-lesion and
                        post-lesion performance (repeated-measure design). Therefore, the additional
                        practice with the WCST, before making the lesions (while they served as the
                        Control group), could not explain the effects of lesions in the OFC or
                        sdlPFC. In the follow up experiments with another cohort of monkeys, we
                        trained 7 macaque monkeys to learn the WCST and then based on individuals’
                        pre-lesion performance (mean number of rule-shifts in each testing session),
                        the monkeys were assigned to two separate groups of matched abilities. One
                        group received bilateral lesions in frontopolar cortex (frontopolar group, n = 4) (Fig. 1b and S 6 ), and the other 3 monkeys did not receive any lesion
                            ( n = 3). In the second stage of this
                        study, the three unoperated monkeys of the second cohort received bilateral
                        selective lesions in the posterior cingulate cortex (PCC) (Fig. 1b and S 7 ). For PCC-lesioned and frontopolar-lesioned animals, we
                        compared RT variability between the pre-lesion and post-lesion performance. The 3 unoperated monkeys performed the WCST while the 15 pre- and 15
                        post-operative testing sessions were completed for the frontopolar-lesioned
                        monkeys. After completion of the post-operative sessions in
                        frontopolar-lesioned monkeys, the 3 unoperated animals received lesions in
                        the PCC. Therefore, the 3 monkeys in the PCC group had more practice with
                        the WCST (compared to the frontopolar-lesioned group). However, as mentioned
                        above, the effects of lesions within the frontopolar cortex or in the PCC
                        were assessed by comparing the pre-lesion and post-lesion performance and
                        therefore, the additional practice with the WCST could not explain the
                        effects of lesions in the frontopolar or PCC groups. Testing and training for cognitive tasks Monkeys were transferred to the experimental room by a
                    transfer-testing cage and positioned in front of a touchscreen. Monkeys could
                    freely move within the testing cage and perform the cognitive task. Open bars at
                    the front of testing cage enabled accessing the touchscreen and a food box in
                    which a food pellet was delivered for correct responses. Monkeys received their
                    daily food in the experimental room. A computer-controlled food box, containing
                    the daily food, was opened at the end of each training/testing session and
                    monkeys were given enough time to access their daily food. Monkeys performed a computerized version of the WCST with the color
                    and shape rules (Fig. 1a ). A set of 36
                    visual stimuli (made of six colors and six shapes) was used in the WCST. In each
                    trial, a sample was selected and presented randomly, without replacement, until
                    all 36 different samples were used and therefore none of the samples was
                    repeated until the entire set was presented in consecutive trials. In each
                    trial, the sample was shown at the center of the touchscreen and after the
                    monkeys touched the sample, then three test items were presented surrounding the
                    sample. One of the test items matched the sample in shape, another test item
                    matched the sample in color and the other test item did not match the sample in
                    either color or shape. Then, monkeys had to select and touch one of the test
                    items that matched the sample according to the relevant rule (matching based on
                    color when color rule was relevant; or matching based on shape when the shape
                    rule was relevant) within a limited response window (3000 ms). A banana-flavored
                    food pellet (190 mg) was provided, as a reward, for each correct response. However, after an erroneous response a visual error signal was presented and no
                    reward was given. In each block of trials, the monkeys had to reach a shift
                    criterion of 17 correct in 20 consecutive trials (85% correct) and then the
                    block changed (a new rule became relevant) without any notification. Monkeys
                    were allowed to perform 300 trials in each daily session. The number of
                    rule-shifts, percentage of corrects and mean response time in correct trials
                    were calculated in each daily testing session. Additional details regarding the
                    setup for training and testing in monkeys and the training steps for the WCST
                    have been reported in our previous publications [25] , [45] , [46] , [85] , [86] . Control behavioral tests In the post-lesion behavioral tests, we also included control tasks
                    in which the rule (color- or shape-matching) remained constant within a daily
                    session (no rule shift was required in the daily testing session). Performance
                    of monkey in all groups (DLPFC, ACC, Control, OFC, sdlPFC, frontopolar and PCC)
                    were comparable and at high level and no group showed any deficit in performing
                    the control tasks. This indicates that monkeys’ sensory, perceptual, motor and
                    attentional abilities remained intact in all experimental
                            groups [25] . Surgery All surgeries were conducted in sterile conditions while monkeys
                    were deeply anaesthetised. On the surgery day, the monkeys were sedated,
                    intubated by a tracheal tube and then connected to an artificial respirator and
                    remained anaesthetized with Isoflurane (1.0−3.0%) during surgery. The same
                    neurosurgeon performed all surgeries at RIKEN institute and Oxford University. All aspiration lesions were visually guided using a surgical microscope. In
                    order to access the target brain region, a bone flap was raised over the left
                    and right prefrontal cortex and then the dura was opened and reflected. Anatomical landmarks were examined to determine the extent of lesion in each
                    animal based on pre-defined criteria. After exposing the brain regions, we used
                    a small-gauge metal aspirator to carefully remove the cortex in the intended
                    brain region. The aspirator was connected to a finely controlled suction system
                    and insulated up to the tip to allow finely targeted electro-cautery. The same
                    procedure was done in the left and right hemispheres. After completion of the
                    lesions in each hemisphere, the dura mater was sewn back and the bone flap was
                    re-positioned and stabilized by dissolvable sutures connected to the skull. The
                    wound was closed and the skin was sewn back. For additional details regarding
                    the surgical approach and pre-operative and post-operative procedures for making
                    selective brain lesions please see our previous
                            publications [25] , [86] . Inactivation studies using chemicals such as GABA agonizts (e.g.,
                    Muscimol) or neurotoxic compounds (e.g., Ibotenic acid) may allow localized
                    inactivation or death of neurons at the injection sites, but cannot mimic the
                    effects of complete disruption of large cortical regions, which were targeted in
                    this study. Increasing the concentration or volume of injections for making
                    complete lesions would cause certain involvement of nearby cortical areas, which
                    would prevent proper interpretation of the lesion effects on cognitive
                    functions. In addition, new molecular-genetic techniques for controlled
                    inactivation/activation of neuronal populations (e.g., DREADD or optogenetics),
                    which have been used in rodent models, are still being developed for
                            primates [87] , [88] . The success rate in transferring the
                    genetic codes to primate neurons is still low and therefore not feasible for
                    complete and bilateral inactivation of deep and large cortical areas, which were
                    targeted in this study. In this study, we used visually-guided aspiration lesion
                    technique, which is still one of the most suitable and currently-available
                    procedure in macaque monkeys to address the goal of this project. Although, the
                    possibility of damage to the immediately underlying white matter cannot be ruled
                    out, we made utmost care during surgery to avoid any deep damage to the
                    underlying white matter and therefore, the possibility of any significant damage
                    to major fascicles was very low. Intended extent of lesions within different brain regions Supplementary figures S6 and S7 include the details of lesion
                    extent for individual monkeys in each lesion group. Anterior cingulate sulcus (ACCs) lesion The extent of intended lesions in the ACC group
                            (Figs. 1b , S 6 ) covered the cortex in the dorsal and
                        ventral banks and depth of the anterior cingulate sulcus, which correspond
                        to cytoarchitectonic areas 24c, 24c’ [35] . The posterior
                        border of the lesion in the cingulate sulcus started at an imaginary line
                        passing through the midpoint of the precentral dimple and the lesion
                        extended anteriorly (rostrally) to include the entire extent of the
                        cingulate sulcus. For the two out of the four ACC-lesioned monkeys, the
                        lesions were complete and as intended, however in another ACC-lesioned
                        monkey the lesion extent was larger than intended in one hemisphere, and in
                        the other monkey, the lesion did not extend as far posteriorly as in the
                        other three monkeys to avoid cutting the ascending branches of the anterior
                        cerebral artery [25] . Dorsolateral prefrontal cortex (DLPFC) lesion The extent of intended lesion in the DLPFC group
                            (Figs. 1b , S 6 ) covered the entire anterior-posterior
                        extent of cortex in both banks and fundus of the principal sulcus. The
                        lesion also extended to surrounding cortical regions 2−3 mm dorsal and
                        ventral to the lips of the principal sulcus on the lateral surface of the
                        prefrontal cortex. Therefore, the DLPFC lesion included the middle portion
                        of cytoarchitectonic areas 46 and 9/46 [35] . Histological
                        examination in two monkeys and 3D structural MRI in the two other monkeys
                        confirmed that the lesion extent was as intended in all four DLPFC-lesioned
                                monkeys [25] . Orbitofrontal cortex (OFC) lesion The extent of intended lesions in the OFC group
                            (Figs. 2b , S 7 ) was limited laterally by the lateral
                        orbital sulcus and therefore included the cortex in the medial bank of the
                        lateral orbital sulcus. The lesion also covered the entire region between
                        the medial and lateral orbital sulci, and extended medially up to the
                        lateral bank of the rostral sulcus. The anterior (rostral) border of the
                        lesion was an imaginary line passing between the anterior tips of the medial
                        and lateral orbital sulci. The posterior limit of the lesions was an
                        imaginary line passing anterior to the posterior tips of the lateral and
                        medial orbital sulci. The intended lesion included the cortex in
                        cytoarchitectonic areas 11, 13 and 14 on the orbital
                                surface [35] . In all three OFC-lesioned monkeys, the
                        lesion covered the intended regions, however in two monkeys there was
                        extremely slight unilateral damage beyond the intended lateral boundary of
                        the lesion and in all three monkeys the lesions did not extent as far
                        medially as intended [25] . Superior dorso-lateral prefrontal cortex (sdlPFC) lesion The extent of intended lesions in the sdlPFC group
                            (Figs. 1b , S 7 ) included the cortex on the most dorsal
                        areas on the lateral prefrontal cortex. The ventral limit of the lesion
                        started 1 mm dorsal to the principal sulcus (Figs. 2 b, 5 ). The
                        lesion extended dorsally up to the longitudinal fissure. Therefore, the
                        lesion included the lateral part of the cytoarchitectonic area 9 and the
                        dorsal portions of areas 46 and 9/46 [35] . However, the
                        lesion did not include the cortex within the principal sulcus area and
                        therefore there was no overlap in the lesion extent between the DLPFC and
                        sdlPFC groups. The lesion extent in the sdlPFC group excluded posteriorly
                        located premotor cortex in cytoarchitectonic areas 8A, 8Bd, and 8Bv, and did
                        not extend to the most anterior regions of prefrontal cortex (did not
                        include area 10) [35] . In the three sdlPFC-lesioned monkeys,
                        the lesion covered the intended regions [25] . Frontopolar cortex lesion The extent of lesions in frontopolar cortex was as intended in
                        all animals and covered the dorsal, medial and orbital parts of frontal pole
                        cortex (Figs. 1b , S 6 ) [65] . The posterior
                        limit of the frontopolar cortex lesions was an imaginary line considered at
                        2 mm posterior to the anterior tip of the principal sulcus. All cortex
                        anterior to this imaginary line was removed. Posterior cingulate cortex (PCC) lesion The extent of lesions in PCC cortex was as intended in all
                        animals and included cortex on the surface of cingulate gyrus (dorsally
                        limited by the cingulate sulcus) and lower bank of posterior cingulate
                        sulcus (Figs. 1b , S 7 ) [65] . The anterior limit
                        of the PCC lesions was an imaginary vertical line at the most posterior
                        level of the central sulcus and the posterior limit was another imaginary
                        line at the most posterior aspect of the splenium of the corpus callosum,
                        which extended to the posterior end of the cingulate sulcus. Histology At the end of data collection, two animals with DLPFC lesion and
                    four animals with ACC lesions were deeply anaesthetized and then perfused
                    through a cannula in the heart with saline and then by formol-saline solution. Animals’ brains were blocked and allowed to sink in sucrose-formalin solution,
                    and subsequently cut in 50 μm sections using a freezing microtome. Every fifth
                    or tenth section was retained and stained with cresyl violet. Histological
                    examination indicated that in all lesion groups the lesion covered the intended
                    cortical regions. The details of lesion extent in each lesion group has been
                    previously reported [25] , [65] . Data analyses Response time (RT) was determined as the interval between the onset
                    of the test items and the first touch of the visual items on the touchscreen
                        (Fig. 1a ). For data analyses, all
                    data points (without removal of any outlier), were used for data analyses. In
                    the WCST, we included a response window for initiating and delivering the
                    response for monkeys and therefore all response times falling outside the
                    response window were considered as errors. Calculation of an index for representing RT variability and
                    comparison between various conditions with different mean RT: The degree of
                    variability might be affected by alterations in the mean RT. Therefore, we
                    calculated Coefficient of RT variation (RT-COV) as the standard deviation of RT
                    divided by the mean RT in each condition [3] , [4] . We used this method to conclude that the
                    variability significantly increased even when the mean RT (significantly or
                    numerically) increased (which is the case in the OFC-lesioned monkeys) (Figs. S 2 and S 5 ), and to conclude that the variability
                    significantly decreased even when the mean RT decreased (which was the case in
                    the ACC-lesioned and DLPFC-lesioned monkeys) (Figs. S 2 and S 5 ). We have
                    also reported the results of statistical tests when standard deviation of RT
                    (SD) was used (Figs. S 1 and
                        S 4 ). As for the effects of lesion
                    on the difference between the RT variability between cE and cC trials, we
                    emphasized the conclusion only when consistent results were obtained with RT-COV
                    and SD. For repeated-measure ANOVA test, Mauchly’s test of sphericity was
                    applied, and if the sphericity was not met, Greenhouse-Geisser corrections were
                    applied. The RT-COV in testing sessions was used as a data point for ANOVA
                    analyses. In all ANOVA analyses, Partial Eta Squared (ηp2) indicates the
                    proportion of the variance explained by the effect, and it was reported for each
                    significant effect. Reporting summary Further information on research design is available in
                        the Nature Portfolio Reporting
                        Summary linked to this article.